Efficient optical extraction of hot-carrier energy Light-induced generation of free charge carriers in semiconductors constitutes the physical basis of photodetection and photovoltaics. To maximize its efficiency, the energy of the photons must be entirely used for this purpose. This is highly challenging owing to the ultrafast thermalization of ‘hot’ carriers, which are created by absorption of high-energy photons. Thermalization leads to heat generation, and hence efficiency loss. To circumvent this, dedicated schemes such as photovoltaic hot-carrier cells are being explored. Here we consider optical extraction of the excess energy of hot carriers by emission of infrared photons, using erbium ions in combination with silicon nanocrystals. We determine the external quantum yield of the infrared photon generation by the erbium ions, and demonstrate that cooling of the hot carriers induces a steep, step-like, increase in erbium-related external quantum yield by up to a factor of 15 towards higher excitation energies. Finally, we comment on the potential of our findings for future photovoltaics in the form of an optical ultraviolet-to-infrared spectral converter. The efficient conversion of the energy of photon is at the heart of many optoelectronic applications and, prominently, detectors and solar cells. For this purpose, new materials and also new physical processes are being explored intensively and considerable progress is being made, with the efficiency of solar cells steadily increasing over the last few decades. In these efforts, a major possibility for further improvement now lies in the (efficient) use of the excess energy of hot carriers. Such carriers are generated by photons whose energies considerably exceed the bandgap of the absorber and their excess energy is typically converted into heat. Harvesting this energy is highly challenging, since thermalization of hot carriers within the host typically takes place on a picosecond time scale or faster. In photovoltaics, heat dissipation by hot carriers constitutes a major loss channel responsible for the Shockley–Queisser efficiency limit [1] , and different strategies to resolve this problem are being explored [2] , [3] , [4] , [5] , [6] , [7] , [8] , [9] . Here we consider an optical approach in which the excess energy of hot carriers is converted into infrared (IR) photons, and in this manner optically extracted to the outside. 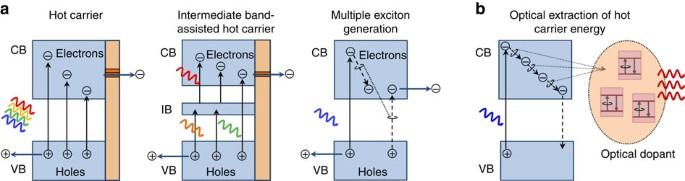Figure 1: Hot-carrier solar-cell concepts. (a) Three currently considered hot-carrier solar-cell strategies: direct extraction of hot carriers through energy-selective contacts, application of an intermediate-band-assisted absorber and using multiple exciton generation, when a hot carrier induces additional excitations across the bandgap. (b) The concept of optical extraction: hot carriers transfer their excess energy to nearby Er3+ions, which subsequently emit IR photons. VB, CB and IB stand for valence, conduction, and intermediate band, respectively. Figure 1 compares the presently considered hot-carrier solar-cell concepts [6] ( Fig. 1a ) with the optical variant described in this work ( Fig. 1b ). The proposed scheme, where absorption of a high-energy photon generates a hot carrier whose cooling results in emission of (multiple) IR photons is conceptually similar to photon cutting with rare-earth (RE) ions [10] , but is much more efficient owing to the participation of silicon nanocrystals (Si NCs). Figure 1: Hot-carrier solar-cell concepts. ( a ) Three currently considered hot-carrier solar-cell strategies: direct extraction of hot carriers through energy-selective contacts, application of an intermediate-band-assisted absorber and using multiple exciton generation, when a hot carrier induces additional excitations across the bandgap. ( b ) The concept of optical extraction: hot carriers transfer their excess energy to nearby Er 3+ ions, which subsequently emit IR photons. VB, CB and IB stand for valence, conduction, and intermediate band, respectively. Full size image The RE-doped materials are frequently investigated for the purpose of light transformation by means of photon down- and upconversion. RE-based phosphors utilizing photon downconversion [10] , [11] , [12] are commonly used in (white) lighting applications, converting ultraviolet photons into the visible range. Upconversion, that is, emission of high-energy photons upon sequential excitation at a lower energy, has also been demonstrated [13] , [14] . However, the common disadvantage of ‘spectral conversion’ with RE ions is their extremely low-absorption cross-section, due to the only marginally allowed character of the optical transitions within the 4f electron shell. To overcome this problem, our approach makes use of thin films of erbium (Er)-doped solid-state dispersions of Si NCs in SiO 2 . In the past, following the interest in Er-doped Si [15] , this material has been intensively investigated so as to develop flash-lamp-pumped optical fibre amplifiers [16] . In this system, the effective excitation cross-section of Er 3+ ions is increased by several orders of magnitude by the energy transfer path from the Si NCs to the Er 3+ ions [17] , [18] , [19] , [20] , [21] . In this case, light initially absorbed by the Si NCs excites the neighbouring Er 3+ ions into the 4 I 13/2 state, which then emit at 0.8 eV. The details of this ‘sensitization’ of Er emission by Si NCs have been thoroughly investigated, and two distinctly different excitation mechanisms have been revealed [19] , [22] : a ‘slow’ one (microseconds), via nonradiative recombination of an electron–hole pair in the ground state, and a ‘fast’ one (sub-nanosecond range), due to intraband cooling transitions of hot carriers. The latter is only available for carriers with a sufficiently large excess energy, and therefore appears exclusively upon absorption of sufficiently energetic photons. In this study, we explore this process for efficient ultraviolet-to-IR conversion with an eye to develop an optical alternative to the photovoltaic schemes presently considered, which are aimed at harvesting the hot-carrier excess energy. External quantum yield of Si NCs- and Er-related PL To investigate the potential of the Si NC-mediated emission from Er 3+ ions for ultraviolet-to-IR spectral conversion, we determined the absolute external quantum yield (EQY, the ratio between the number of emitted and absorbed photons) of Er-related photoluminescence (PL) in differently prepared materials—see Methods for a description of the experimental setup for EQY determination and characteristics of the samples used in the study. 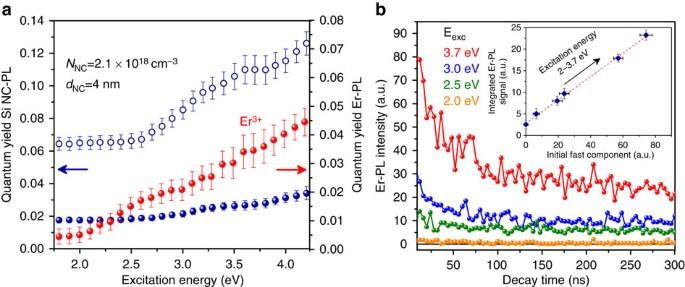Figure 2: EQY of Si NC- and Er-related PL together with hot-carrier-mediated Er excitation. (a) EQY of Si NC- (blue) and Er-related (red) PL from undoped (open circles) and Er-doped (solid circles) samples. Both samples have the similar average NC diameterdNC=4 nm and concentrationNNC=2.1 × 1018cm−3. (b) Decay dynamics of 0.8 eV Er-related emission for the first 300 ns after the excitation pulse, normalized to an equal (and low, below saturation) photon flux. The fast component appears for above-threshold excitations and increases with higher energies. The inset shows the integrated Er-related emission at 0.8 eV as a function of the initial amplitude of the fast decaying signal. Figure 2a presents a comparison of EQY of Si NC- and Er-related emission bands in Er-doped and Er-free samples as a function of excitation photon energy. Both samples have identical average diameter ( d NC ) and concentration of Si NCs ( N NC ) of 4 nm and 2.1 × 10 18 cm −3 , respectively, see Supplementary Fig. 1 , for the emission spectra of these samples. The NC-related PL in the undoped sample has a constant EQY of ~6.5% for excitation energies below ~2.5 eV (about twice the bandgap energy), and increases in a step-like manner above this threshold. In the past, this behaviour has been investigated in detail and is assigned to the specific carrier multiplication (CM) process [23] , which increases the number of excitons generated by absorption of a single photon with a sufficiently high energy [24] , [25] . Upon doping with Er 3+ ions, the EQY of NC-related PL is reduced while its excitation dependence remains similar, indicating that although the relevant CM process is still active, the PL efficiency of the NCs is reduced. This is readily understood, since in the doped sample a part of the NCs, which previously contributed to PL, now excite neighbouring Er 3+ ions. Further, we note that the EQY of the Er-related PL also shows a threshold-governed increase, but with the threshold energy significantly lower than that for CM. The increase of EQY from the initial value of ~0.5% appears to be due to the onset of the hot-carrier-mediated Er 3+ -ion excitation process, which operates at higher pump energies, in addition to the slow exciton energy transfer [24] . The threshold for this is given by the sum of the bandgap energy of Si NCs and the 0.8 eV energy of the 1st excited state of Er 3+ ion, and in this particular material appears at E 1 =2.0–2.1 eV. For the highest investigated pump photon energy of 4.25 eV, the EQY of Er-related PL reaches ~4.5%. Figure 2: EQY of Si NC- and Er-related PL together with hot-carrier-mediated Er excitation. ( a ) EQY of Si NC- (blue) and Er-related (red) PL from undoped (open circles) and Er-doped (solid circles) samples. Both samples have the similar average NC diameter d NC =4 nm and concentration N NC =2.1 × 10 18 cm −3 . ( b ) Decay dynamics of 0.8 eV Er-related emission for the first 300 ns after the excitation pulse, normalized to an equal (and low, below saturation) photon flux. The fast component appears for above-threshold excitations and increases with higher energies. The inset shows the integrated Er-related emission at 0.8 eV as a function of the initial amplitude of the fast decaying signal. Full size image Hot-carrier-mediated Er excitation According to the proposed interpretation, the EQY enhancement of Er-related PL at higher energies is attributed to the hot-carrier-mediated excitation route. The contribution of this mechanism to the total PL signal can be directly evaluated from the initial fast-decay component in the Er-PL dynamics, that is, within the first microsecond after the pump pulse [19] . Figure 2b illustrates the initial decay dynamics, experimentally measured for several values of excitation energy, normalized to an equal (and low) photon flux. As can be seen, the fast decaying component indeed appears for above-threshold pumping and then increases at still higher energies, see Supplementary Fig. 2 for an illustration of a complete decay dynamics of the Er-related PL. While the majority of Er 3+ ions excited by hot carriers quench rapidly by a reverse Auger process of energy transfer back to Si NCs, some escape the quenching and de-excite radiatively, thus contributing to the slowly decaying Er-PL signal. In the inset of Fig. 2b , we plot the total time-integrated Er-PL signal as a function of the initial amplitude of the fast component; evidently, a linear dependence is obtained, confirming the proposed identification. Interestingly, we note that the PL intensity does not increase from zero. This initial value represents the PL contribution from the slow excitation mechanism, which is due to electron–hole recombination. For completeness, we also investigated the power dependence of the Er-PL: a linear dependence has been obtained, with a slope corresponding to the EQY at the particular excitation energy—see the inset in Supplementary Fig. 2 for a typical dependence, as obtained for a high-energy pumping (E exc =3 eV), where both excitation mechanisms are active. Material optimization To explore the potential of the energy transfer to Er 3+ ions as an effective route for extraction of excess energy from hot carriers, we investigated how the EQY of Er-related PL changes with the material characteristics. 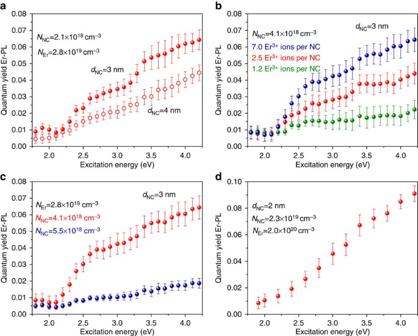Figure 3: EQY dependence on material characteristics. (a)EQY of Er-related PL from samples with a NC diameter ofdNC=3 nm (solid red circles) anddNC=4 nm (open red circles). (b) The comparison of the EQY of three samples having different Er3+ion concentrations but the same Si NC size and concentration. The enhancement of the EQY at higher excitation energies increases with the Er concentration. (c) Comparison of EQY of two samples having same Er3+ion concentration and Si NCs size but different Si NC concentration. The enhancement of EQY decreases with increasing Si NC concentration. (d) EQY of sample with a NC diameter ofdNC=2 nm and a high concentration of Er3+ions, showing ~15-fold increase in EQY over the investigated excitation energy range. Figure 3a compares the EQY of the Er-related PL in two samples with identical concentrations of Er and Si NCs, but with different average NC diameters, namely d NC =3 nm and d NC =4 nm. For both samples a threshold-governed enhancement is observed, marking the transition between the energy regimes for which single and multiple Er 3+ ions excitations can be accomplished on absorption of a single photon. The threshold energy seems somewhat higher for smaller NCs, which we attribute to their larger bandgap. We note that for this sample also the initial EQY is higher and, again, rises for larger pump energies. Peculiarities that can be noted in the experimentally determined dependence of EQY (‘steps’) possibly mark subsequent thresholds, as the growing excess energy enables excitation proceeding to multiple Er 3+ ions and/or higher excited states. To this end, we recall that a step-like increase of efficiency on Er concentration has also been reported for energy transfer between Er 3+ ions in erbium silicide [12] . Figure 3: EQY dependence on material characteristics. ( a )EQY of Er-related PL from samples with a NC diameter of d NC =3 nm (solid red circles) and d NC =4 nm (open red circles). ( b ) The comparison of the EQY of three samples having different Er 3+ ion concentrations but the same Si NC size and concentration. The enhancement of the EQY at higher excitation energies increases with the Er concentration. ( c ) Comparison of EQY of two samples having same Er 3+ ion concentration and Si NCs size but different Si NC concentration. The enhancement of EQY decreases with increasing Si NC concentration. ( d ) EQY of sample with a NC diameter of d NC =2 nm and a high concentration of Er 3+ ions, showing ~15-fold increase in EQY over the investigated excitation energy range. Full size image From the data presented in Fig. 3a , we note that both the absolute value as well as the enhancement of EQY through the hot-carrier-mediated excitation depends on the sample characteristics. For the material with d NC =4 nm, this contribution is ~4% (boosting the EQY from ~0.5 to ~4.5%), and ~5.5% for d NC =3 nm (from ~1 to ~6.5%). To further explore the EQY dependence on material characteristics, we investigated the EQY of Er-related PL on changes in the absolute concentrations of Si NCs and Er 3+ ions, N NC and N Er , respectively, as well as their relative ratios. The results are illustrated in Fig. 3b for different N Er (identical d NC and N NC ) and in Fig. 3c for different N NC (identical d NC and N Er ). In all cases a similar threshold-governed increase in EQY is observed, with the initial value of the EQY at low energies being determined by the slow energy transfer, and the subsequent enhancement by the hot-carrier-mediated excitation. From these we conclude that to maximize the energy extraction from hot carriers by Er 3+ emission (i) the ratio of N Er / N NC should be high and (ii) a smaller diameter of NCs, d NC , is preferred. The EQY for a sample prepared according to these preliminary and crude guidelines (with d NC =2 nm, N NC =2 × 10 19 cm −3 , N Er =2 × 10 20 cm −3 ) is depicted in Fig. 3d . We conclude that in this case practically 9% of the EQY is induced by the hot-carrier energy, leading to ~15-fold increase over the investigated excitation range. As can be concluded from the presented data, within the investigated energy range, the EQY of the IR Er-related emission increases by an order of magnitude due to hot-carrier-mediated excitation. At the same time, the maximum excess energy with respect to the threshold is in this study 4.25 eV−(~2.1 eV)≈2.15 eV. With the energy of the first excited state of Er being 0.8 eV, this allows for an excitation of on average at maximum of 2.5 additional Er 3+ ions per absorbed photon. Therefore, the much larger increase of the EQY implies that many more Si NCs can take part in the hot-carrier-mediated excitation than in the exciton-mediated one. This conclusion is consistent with the much faster dynamics of this process, which apparently successfully competes with other channels through which the hot carriers can lose energy. We note that the EQY of ~9% for excitation at 4.25 eV shown in Fig. 3d implies that we get 9 photons of energy 0.8 eV per absorption of 100 photons of energy 4.25 eV. In absolute terms, we thus optically extract 7.2 eV energy per 245 eV of excess energy of the hot carrier generated in Si NCs with a bandgap of 1.8 eV. This therefore gives an experimentally demonstrated net external energy extraction efficiency (energy of the emitted photon divided by the energy of the absorbed photon) of 3%. Finally, we comment on a possible application potential of the presented findings for photovoltaics. We note that the spectral transformation process considered here represents an optical equivalent of multiple carrier generation at the optimal energy of 0.8 eV; the theoretical limit of the conversion efficiency is in this case close to 45% [26] , considerably above the Shockley–Queisser limit. A thin, optimized, active layer of SiO 2 doped with Si NCs and Er 3+ ions could be added to a solar cell or integrated into, for example, the antireflective coating. This layer would absorb photons of the highest energy, whose conversion efficiency in a Si cell is the lowest, ‘cut’ them into multiple IR photons and direct them into an appropriate photovoltaic device. Such a ‘solar shaper’ would then allow the harvesting of a portion of the excess energy of photogenerated carriers—energy that is typically converted to heat in the standard solar cell. By adjusting the size and concentration of Si NCs, the Er 3+ ion concentration and the thickness of the active layer, the absorbance in the active layer can be tuned to optimize the division of the solar photon flux. In conclusion, we have determined the EQY for the conversion of ultraviolet-to-IR photons by Er 3+ ions in SiO 2 layers doped with Si NCs. Investigating the dependence of the EQY for IR emission on the primary photon energy, we show a steep growth in EQY, yielding an up to ~15-fold enhancement of EQY for high-excitation photon energies. This appears to be due to efficient energy transfer between hot carriers in the Si NCs and multiple neighbouring Er 3+ ions in the SiO 2 matrix. This energy conversion process offers a promising path for an optical extraction of the excess energy of hot carriers. Future material engineering will show whether the currently demonstrated maximal EQY of 9% can be sufficiently increased, so as to allow its practical application for ultraviolet-to-IR photovoltaic shapers. Samples The investigated ~2-μm-thick layers containing Si NCs with Er 3+ ions in SiO 2 have been fabricated on a quartz substrate using a radio-frequency co-sputtering technique. The sputtering procedure was followed by an annealing step for 30 min in a N 2 atmosphere. After annealing, the samples were characterized by Si NCs sizes, concentrations of Si NCs and Er 3+ ions and thereby divided into four categories: i Two samples having the same concentration of Si NCs ( N NC =2.1 × 10 18 cm −3 ) and Er 3+ ions ( N Er =2.8 × 10 19 cm −3 ) but different average Si NCs sizes of d NC =3 nm and d NC =4 nm following annealing at 1,100 and 1,200 °C, respectively. ii Three samples annealed at 1,100 °C with the same Si NCs concentration of N NC =4.1 × 10 18 cm −3 and size d NC =3 nm but with different Er 3+ ion concentration of N Er =0.5 × 10 19 , 1.1 × 10 19 and 2.8 × 10 19 cm −3 . iii Two samples with the same Er 3+ ion concentrations N Er =2.8 × 10 19 cm −3 and NCs size of d NC =3 nm but different Si NC concentrations of N NC =2.1 × 10 18 and 5.5 × 10 18 cm −3 , both samples being annealed at 1,100 °C. iv One sample with a higher Er 3+ ion concentration of N Er =2.0 × 10 20 cm −3 , and Si NCs concentration of N NC =2.3 × 10 19 cm −3 and d NC =2 nm. PL and decay time measurements Measurements of PL spectra were performed under continuous wave excitation with Nd:YVO 4 laser (Millennia, Spectra Physics), operating at 532 nm. The PL signal was recorded with a 1-m f/8 monochromator (Jobin-Yvon THR-1000) coupled to an IR Ge detector (Edinburgh Instruments) with a DSP lock-in amplifier (Signal Recovery SR7265). The results were corrected for the spectral response of the system. A photomultiplier tube (Hamamatsu R5509-73, 300–1,700 nm) working in the time-correlated single-photon-counting mode, coupled to a 1-m f/8 monochromator was used to measure the PL life time. These measurements were performed under pulsed excitation at different energies by making use of a tunable optical parametric oscillator pumped by the third harmonic of a Nd:YAG laser, with the pulse duration of ~10 ns and the repetition rate of 100 Hz. EQY measurements The EQY of the PL is defined as the ratio of the number of emitted photons (integrated PL signal, corrected for that of the SiO 2 substrate only) to the number of absorbed photons (integrated decrease of the excitation). The measurements of the EQY were performed using an integrating sphere, under excitation by a 150-W xenon lamp (Hamamatsu L2273) coupled to a double-pass monochromator (Solar MSA-130). To calculate the number of absorbed photons, the spectra of different excitation energies were recorded by placing the reference (quartz substrate) and the investigated samples in the integrating sphere. From the difference between excitation spectra recorded for the sample and the reference, the absorption in the Si NC layer was obtained. This was done by making use of a monochromator (Solar M266) coupled to a charge coupled device (Hamamatsu S10141-1108S, 200–1,100 nm). The 0.8 eV emission signal from the Er 3+ ions was recorded using a Ge detector (Edinburgh Instruments) together with lock-in amplifier (Signal Recovery SR 7265). All the measurements were corrected for the spectral response of the systems. Since the absorption and emission signals were recorded using two different detection systems, it was important to correctly scale their efficiencies. For details of the scaling procedure see Supplementary Methods . How to cite this article: Saeed, S. et al . Efficient optical extraction of hot-carrier energy. Nat. Commun. 5:4665 doi: 10.1038/ncomms5665 (2014).